Haemogenic endocardium contributes to transient definitive haematopoiesis Haematopoietic cells arise from spatiotemporally restricted domains in the developing embryo. Although studies of non-mammalian animal and in vitro embryonic stem cell models suggest a close relationship among cardiac, endocardial and haematopoietic lineages, it remains unknown whether the mammalian heart tube serves as a haemogenic organ akin to the dorsal aorta. Here we examine the haemogenic activity of the developing endocardium. Mouse heart explants generate myeloid and erythroid colonies in the absence of circulation. Haemogenic activity arises from a subset of endocardial cells in the outflow cushion and atria earlier than in the aorta-gonad-mesonephros region, and is transient and definitive in nature. Interestingly, key cardiac transcription factors, Nkx2–5 and Isl1, are expressed in and required for the haemogenic population of the endocardium. Together, these data suggest that a subset of endocardial/endothelial cells serve as a de novo source for transient definitive haematopoietic progenitors. The circulatory system is the first functional organ system that develops during mammalian life. The heart tube is a highly modified muscular vessel that starts to beat even prior to its connection with the dorsal aortae, and yet shares a common genetic program with the dorsal aorta and other arteries [1] . The dorsal aorta is, however, not merely a conduit, but also a source for the third component of the circulatory system, the blood cells. During mammalian embryogenesis, haematopoiesis occurs in several major anatomical sites, including the yolk sac, placenta and the aorta-gonad-mesonephros (AGM) region that contains the dorsal aorta [2] , [3] , [4] , [5] . A common feature of these known de novo haemogenic sites is that the induction and generation of definitive haematopoietic cells is closely associated with the arterial differentiation [6] , [7] , [8] , [9] , [10] , [11] . Haemodynamic stress and local nitric oxide also have a critical role in haematopoietic induction from the endothelium [10] , [11] . The endocardium shares all these properties with arterial endothelium, including the arterial marker expression and exposure to the haemodynamic stresses and nitric oxide. However, despite all the structural, molecular and haemodynamic similarities between the heart tube and the dorsal aorta, little is known about the haemogenic potential of the endocardium. We have previously demonstrated that cardiac and endocardial/endothelial cells can arise from a single common progenitor cell expressing Flk1, Isl1 and Nkx2–5 during early mammalian cardiogenesis [12] . Notably, these early cardiac progenitors express multiple haematopoietic transcription factors, consistent with previous reports [13] . However, the biological significance of haematopoietic genes in the developing mammalian heart is unknown: this may represent a transient programme that is subsequently repressed [14] . Alternatively, as in the dorsal aorta, a haematopoietic programme may be activated in the heart. As a close relationship among cardiac, endocardial and haematopoietic lineages has been suggested in fly, zebrafish and embryonic stem cell in vitro differentiation models [15] , [16] , [17] , [18] , [19] , [20] , critical questions are when, where and how this haematopoietic gene programme is in operation during in vivo mammalian cardiogenesis. Here, we report the haemogenic activity of the endocardium in developing mammalian heart and its Nkx2–5/Isl1-dependent mechanism. The early heart tube is a de novo site for haematopoiesis Defining the origin of blood cells in vivo is complicated by circulation. Once an effective heartbeat is initiated at around 8 somite stage (~E8.5), any blood cell may circulate and adhere to any vascular wall throughout the body. To examine whether the heart tube generates functional haematopoietic cells in situ , we employed two methods. First, we examined the colony-forming activity of the heart tubes explanted at pre-circulation stages (1–5 somite stages) on an OP9 feeder layer, which supports myelo-erythroid differentiation [21] , followed by methylcellulose culture supplemented with haematopoietic growth factors ( Fig. 1a ). As a positive control, yolk sac yielded numerous colonies ( Fig. 1b ). The caudal half of the embryo (including dorsal aortae) and allantois (future placenta) also produced a much smaller but significant number of colonies, and the head explants produced no colonies at any stages. Interestingly, the heart tubes explanted from pre-circulation stages developed erythroid, myeloid and mixed lineage clonogenic progenitors ( Fig. 1b ). Second, to further confirm the in situ haemogenic activity of the heart tube, we utilized the Ncx1 -knockout mouse model. Ncx1 is a sodium–calcium exchanger, of which expression is restricted to the myocardium. Ncx1 -mutant embryos show normal morphogenesis and cardiac gene expression until E9.5, but do not survive after E10.5 (ref. 22 ). They have no heartbeat, and thus no systemic circulation, which makes them a suitable model for examining local haematopoietic emergence [22] . OP9 coculture and subsequent colony assays revealed that the heart explants from Ncx1 mutants at E9.5 generated blood colonies in the absence of effective circulation ( Fig. 1c ). Together, these experiments suggest that the heart tube displays in situ haemogenic activity during embryogenesis. 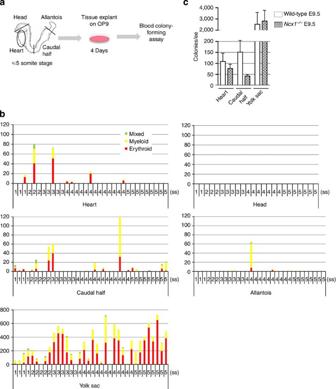Figure 1: The heart tube is ade novosource for haematopoietic cells. (a) Schematic representation of the colony-forming assay fromex vivoorgan explant at pre-circulation stages. The heart tube, head, allantois, caudal half (including future AGM region) and yolk sac were dissected at somite stages 1–5, before the formation of effective circulatory loop. Tissues were washed in three changes of PBS and cultured on an OP9 feeder layer for 4 days, followed by methylcellulose culture in the presence of haematopoietic growth factors. (b) Haematopoietic colonies retrieved from various tissues at various somite stages. Each column represents colonies from one tissue. The heart tubes displayed haematopoietic activity whereas the head explants did not. Note the difference in the scale in the yolk sac. (c) Colonies fromNcx1-mutant embryos that lack heartbeat, showing the haematopoietic activity in the heart tube in the absence of effective heartbeat. ee; embryo equivalent. Mean±s.e.m. Figure 1: The heart tube is a de novo source for haematopoietic cells. ( a ) Schematic representation of the colony-forming assay from ex vivo organ explant at pre-circulation stages. The heart tube, head, allantois, caudal half (including future AGM region) and yolk sac were dissected at somite stages 1–5, before the formation of effective circulatory loop. Tissues were washed in three changes of PBS and cultured on an OP9 feeder layer for 4 days, followed by methylcellulose culture in the presence of haematopoietic growth factors. ( b ) Haematopoietic colonies retrieved from various tissues at various somite stages. Each column represents colonies from one tissue. The heart tubes displayed haematopoietic activity whereas the head explants did not. Note the difference in the scale in the yolk sac. ( c ) Colonies from Ncx1- mutant embryos that lack heartbeat, showing the haematopoietic activity in the heart tube in the absence of effective heartbeat. ee; embryo equivalent. Mean±s.e.m. Full size image CD41 is expressed in a subset of the endocardial cells We hypothesized that the de novo haematopoietic activity of the heart tube arises from endocardium because it shares many of the properties with the endothelium in the dorsal aorta. To examine the haemogenic potential of the endocardium, we first analysed the local expression of CD41 (integrin alpha2b, GpIIB), an early surface marker for nascent haematopoietic progenitor cells. Immunostaining revealed that CD41 is expressed in a subset of CD31 + endocardial cells in the outflow tract and atria ( Fig. 2a , arrows). CD31 + /CD41 + endocardial cells were rounded up and scattered circumferentially in atria and less frequently in ventricles. Clusters of CD31 + /CD41 + cells were found in the endocardial cells in the outflow cushion, atrioventricular (AV) cushion, aortic sac, aortic arches and the dorsal atrial wall near the dorsal mesocardium where the common atrial chamber and future pulmonary vein are in the process of establishing a connection ( Supplementary Fig. S1 ). CD41 + cells were identified even at E8.25 in the endocardium, but not until around E10.5 in the AGM ( Supplementary Fig. S2 ), indicating that the CD41 + putative haematopoietic progenitor cells emerge earlier in endocardium than in the endothelium of the AGM. Although CD41 also labels megakaryocytes/platelets, the majority of CD41 + cells in the endocardium were non-megakaryocyte/platelets at these stages, as they were negative for GP1bβ ( Supplementary Fig. S3 ). Co-staining using an antibody against phosphorylated histone H3 (pH3) suggests that CD31 + /CD41 + cells proliferate in situ on the endocardial wall ( Supplementary Fig. S4 ). Furthermore, electron microscopic analysis of the embryonic hearts at E9.5–10.5 revealed that some of the endocardial cells are rounded up ( Fig. 2c , middle panels) and protrude into the cardiac lumen ( Fig. 2c , right panels). These cells have relatively large nuclei, and are connected to adjacent endocardial cells by adherens junctions ( Fig. 2c , bottom panels), suggesting that they are not circulating blood cells attaching to the endocardial wall, but are endocardial cells emerging into circulation. Together, these data indicate that these putative haematopoietic progenitors are generated in situ in the endocardium. 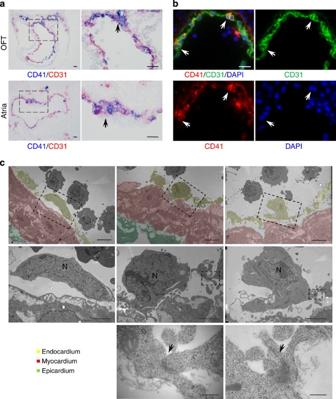Figure 2: A subset of endocardial cells express CD41 and undergo budding into the heart lumen. (a) Immunohistochemistry for CD41 (blue) and CD31 (red) in outflow tract (OFT) and atria at E9.5. CD41+endocardial cells are clustered in the outflow cushion and the dorsal wall of the atria, and also scattered in the entire circumference (arrows). Scale bar, 100 μm (lower magnification), 50 μm (higher magnification). (b) Immunofluorescent staining for CD41 (red), CD31 (green) and DAPI (blue) in left atrium at E9.5. Arrows indicate scattered CD31+endocardial cells co-expressing CD41. Scale bar, 20 μm. (c) Electron microscopic analysis of E10.0–10.5 atrium. Bottom panels show higher magnification of the broken-lined area in upper panels. Left panels indicate regular flat endocardial cells. Centre panels are representative images of endocardial cells rounded up. Endothelial cells occasionally protrude into the cardiac lumen (right panels). The bottom panels are higher magnification of adherens junctions in the dotted area in the middle panels (arrows). Scale bar, 2 μm (upper panels), 1 μm (middle panels) and 100 nm (bottom panels). Yellow, endocardial layer; red, myocardial layer; N, nucleus. Figure 2: A subset of endocardial cells express CD41 and undergo budding into the heart lumen. ( a ) Immunohistochemistry for CD41 (blue) and CD31 (red) in outflow tract (OFT) and atria at E9.5. CD41 + endocardial cells are clustered in the outflow cushion and the dorsal wall of the atria, and also scattered in the entire circumference (arrows). Scale bar, 100 μm (lower magnification), 50 μm (higher magnification). ( b ) Immunofluorescent staining for CD41 (red), CD31 (green) and DAPI (blue) in left atrium at E9.5. Arrows indicate scattered CD31 + endocardial cells co-expressing CD41. Scale bar, 20 μm. ( c ) Electron microscopic analysis of E10.0–10.5 atrium. Bottom panels show higher magnification of the broken-lined area in upper panels. Left panels indicate regular flat endocardial cells. Centre panels are representative images of endocardial cells rounded up. Endothelial cells occasionally protrude into the cardiac lumen (right panels). The bottom panels are higher magnification of adherens junctions in the dotted area in the middle panels (arrows). Scale bar, 2 μm (upper panels), 1 μm (middle panels) and 100 nm (bottom panels). Yellow, endocardial layer; red, myocardial layer; N, nucleus. Full size image Endocardial cells display haemogenic activity To examine haemogenic activity of the endocardium, we performed a blood colony-forming assay using fluorescence-activated cell sorting (FACS)-purified endocardial/endothelial cells from embryonic tissues as previously described [23] , [24] . As a subset of circulating haematopoietic progenitor cells express CD31, the local endocardial cells at E9.5 and 10.5 were sorted as a CD31 + /CD41 − /CD45 − population ( Supplementary Fig. S5a ). The CD31 + /CD41 − /CD45 − cell population in the heart at these stages represents endocardial cells, as coronary vessels are not yet formed. Microarray analysis from CD31 + /CD41 − /CD45 − cells in the heart, caudal half and yolk sac identified 23,922 gene probes expressed in the endocardium, 19,387 of which are expressed in common and 1,829 of which are specific to the endocardium ( Supplementary Fig. S5b ). The CD31 + /CD41 − /CD45 − population of the endocardium shared expression of haematopoietic genes with other endothelial populations, including Cbfa2t3 , Kit , Klf1 , Mll1 , Pbx1 and Scl / Tal1 ( Supplementary Fig. S5c , Supplementary Table S1 ). Within 20,966 gene probes commonly expressed in the heart tube and caudal half, 4,631 probes were expressed within 1.5-fold from each other. These similarly expressed probes included 481 transcription factors ( Supplementary Table S2 ). Gene ontology analyses of these probe sets showed that haematopoiesis-related transcription factors are significantly enriched in this group ( Supplementary Fig. S5d ). PCR suggests that Runx1 , cMyb , Klf1 and Scl are expressed in the endocardium ( Supplementary Fig. S5e ). As non-haemogenic tissue is not included in the analysis, it is possible that all the endothelial cells at this stage express some level of haematopoietic transcription factors. However, colony assays with OP9 coculture revealed that myeloid colonies and rare erythroid colonies develop from FACS-purified endocardium ( Supplementary Fig. S6a , b, d). Direct colony assay without OP9 preculture yielded no colony from the heart or AGM ( Supplementary Fig. S6c ), indicating that CD31 + /CD41 − /CD45 − cells are not yet committed to the haematopoietic progenitor fate and that there is no contamination of circulating haematopoietic progenitors with this sorting method. Together, these data suggest that the endocardium is capable of generating functional haematopoietic cells ex vivo , and support the idea that endocardium is a novel site of de novo haematopoiesis in the developing embryo. CD41 + endocardial cells arise from Nkx2–5 + cells One of the few genes known to be differentially expressed in the endocardium is a homeobox transcription factor, Nkx2–5 [25] , [26] . Previous reports suggest that Nkx2–5 + cells contribute to the endocardial cells and that Nkx2 – 5 messenger RNA is expressed in the endocardium [25] , [26] . While the function of Nkx2–5 in the myocardium is extensively studied, little is known about its function in the endocardium/endothelium [26] . Immunostaining revealed that Nkx2–5 is expressed in a subset of endocardial cells in the outflow and AV cushion, the dorsal wall of the atria and the aortic sac, although the expression level was significantly weaker than that in the myocardium ( Fig. 3a ). Consistently, lineage tracing using Nkx2 – 5 IRES-Cre/+ ; R26 YFPR/+ showed clusters of YFP + cells in the outflow cushion endocardium ( Fig. 3b , upper panels) and the atrial endocardium near the dorsal mesocardium ( Fig. 3b , lower panels). Isolated YFP + cells were also found scattered in other parts of the atrial and outflow endocardium. As this specific distribution pattern of Nkx2–5-positive/-derived cells corresponded to that of CD31 + /CD41 + cells in the endocardium ( Fig. 2a ,b, and Supplementary Fig. S1 ), we examined whether CD41 is expressed in YFP + cells in the endocardium. Double staining for YFP/CD41 in Nkx2 – 5 IRES-Cre/+ ; R26 YFPR/+ hearts revealed that the majority of endocardial CD41 + cells arise from Nkx2–5-derived endocardium ( Fig. 3c ). These data suggest that Nkx2–5-positive endocardium represents the haemogenic subpopulation in the endocardium. Nkx2–5-positive/-derived cells are also found in the yolk sac endothelium with variation in frequency, but not in the AGM endothelium ( Supplementary Fig. S7 ). 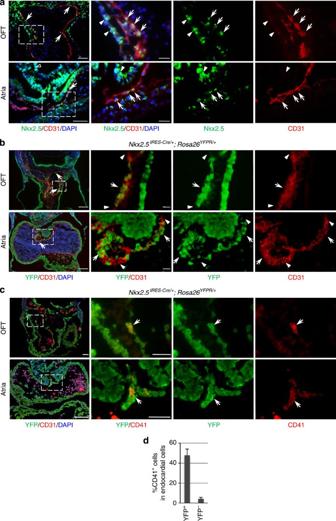Figure 3: Expression of CD41 in Nkx2–5-positive subset of endocardial cells. (a) Immunofluorescent staining for Nkx2–5 (green) and CD31 (red) at E9.5. Clusters of Nkx2–5+cells are found in the endocardium of outflow cushion, AV cushion and the dorsal wall of the atria (white arrows). Note that myocardium shows stronger level of Nkx2–5 expression (white arrowheads). Endodermal cells are also positive for Nkx2–5 (left lower panel, open arrowhead). Scale bar, 50 μm (lower magnification), 20 μm (higher magnification). (b) Heart section ofNkx2–5IRES-Cre/+; R26YFPR/+embryo at E10.5 stained for YFP (green) and CD31 (red). Nkx2–5-derived endocardial cells (YFP/CD31 double positive) were clustered in the outflow cushion and the dorsal wall of the atrium, and also found scattered along the perimeter (arrows). This specific distribution pattern corresponds to that of CD41+cells (Fig. 2a). Arrowheads indicate non-Nkx2–5-derived endocardial cells. Scale bar, 100 μm (lower magnification), 20 μm (higher magnification). (c) Heart section ofNkx2–5IRES-Cre/+; R26YFPR/+embryo at E10.5 stained for YFP (green) and CD41 (red). Nkx2–5+cells give rise to CD41+cells in the endocardium (YFP/CD41 double positive, arrows). Scale bar, 100 μm (lower magnification), 20 μm (higher magnification). (d) Percentage of CD41+cells in Nkx2–5-derived fraction of endocardium at E9.5. 48% of Nkx2–5-lineage-labelled endocardial cells express CD41 whereas 4.4% are CD41-positive in non-Nkx2–5-derived endocardial cells. The graph represents the average of three independent experiments. Mean±s.e.m. Figure 3: Expression of CD41 in Nkx2–5-positive subset of endocardial cells. ( a ) Immunofluorescent staining for Nkx2–5 (green) and CD31 (red) at E9.5. Clusters of Nkx2–5 + cells are found in the endocardium of outflow cushion, AV cushion and the dorsal wall of the atria (white arrows). Note that myocardium shows stronger level of Nkx2–5 expression (white arrowheads). Endodermal cells are also positive for Nkx2–5 (left lower panel, open arrowhead). Scale bar, 50 μm (lower magnification), 20 μm (higher magnification). ( b ) Heart section of Nkx2 – 5 IRES-Cre/+ ; R26 YFPR/+ embryo at E10.5 stained for YFP (green) and CD31 (red). Nkx2–5-derived endocardial cells (YFP/CD31 double positive) were clustered in the outflow cushion and the dorsal wall of the atrium, and also found scattered along the perimeter (arrows). This specific distribution pattern corresponds to that of CD41 + cells ( Fig. 2a ). Arrowheads indicate non-Nkx2–5-derived endocardial cells. Scale bar, 100 μm (lower magnification), 20 μm (higher magnification). ( c ) Heart section of Nkx2 – 5 IRES-Cre/+ ; R26 YFPR/+ embryo at E10.5 stained for YFP (green) and CD41 (red). Nkx2–5 + cells give rise to CD41 + cells in the endocardium (YFP/CD41 double positive, arrows). Scale bar, 100 μm (lower magnification), 20 μm (higher magnification). ( d ) Percentage of CD41 + cells in Nkx2–5-derived fraction of endocardium at E9.5. 48% of Nkx2–5-lineage-labelled endocardial cells express CD41 whereas 4.4% are CD41-positive in non-Nkx2–5-derived endocardial cells. The graph represents the average of three independent experiments. Mean±s.e.m. Full size image Nkx2–5 + cells contribute to definitive haematopoiesis To characterize the developmental nature of Nkx2–5-derived haematopoietic population, we first examined the contribution of Nkx2–5 + cells to the peripheral circulation. Examination of the peripheral blood in Nkx2 – 5 IRES-Cre/+ ; R26 YFPR/+ embryos identified YFP-labelled cells in the circulating blood ( Fig. 4a , upper panels, arrows). YFP-labelled CD45 + cells also repopulated the liver ( Fig. 4a , lower panels, arrows). FACS analysis of the peripheral blood in Nkx2 – 5 IRES-Cre/+ ; R26 YFPR/+ embryos revealed that Nkx2–5 + cells contributed to 4% of peripheral Ter119 + (erythroid) cells and 12% of peripheral CD45 + (non-erythroid) cells at E10.5. At E15.5, the percentage of Nkx2–5-derived Ter119 + and CD45 + became 2.9% and 0.1%, respectively ( Fig. 4b ). However, Nkx2–5-derived blood cells were not identified in the peripheral circulation in adult Nkx2 – 5 IRES-Cre/+ ; R26 YFPR/+ mice. Expression analysis by quantitative PCR (qPCR) for β-globin genes indicates that Nkx2–5-derived erythroids were initially positive for Hbb-bh1 and Ey at E10.5, and underwent maturational globin switching to Hbb-b1 and Hbb-b2 by E15.5 ( Fig. 4c ). FACS analyses of E9.5 Nkx2 – 5 IRES-Cre/+ ; R26 YFPR/+ embryos suggested that about 16% and 7.5% of CD41 + /c-kit + cells in the heart and the yolk sac, respectively, were derived from Nkx2–5 + cells ( Supplementary Fig. S8 ). To examine whether Nkx2–5 + cells contribute to the definitive erythroids, circulating Ter119 + cells were separated using forward and side scatter [27] . Hoechst staining from primitive (P2) and definitive (P1) erythroids showed distinct nucleated and enucleated cells ( Fig. 4d ) as previously demonstrated [27] . As shown in the upper the panels of Fig. 4d , Nkx2–5 + cells contributed to both primitive nucleated and definitive enucleated cells. qPCR from YFP + nucleated primitive and YFP + enucleated definitive erythroids showed a typical Hbb-Ey and Hbb-b1/b2 dominant pattern of β-globin expression, respectively ( Fig. 4d , bottom panel). Furthermore, analyses of Runx1 mutants ( Runx1 lz/rd ) revealed that Runx1 is required for the formation of haematopoietic colonies, although not for the specification of CD41 + cells in the endocardium ( Supplementary Fig. S9 ). Together, these data suggest that Nkx2–5 + haemogenic endocardial/endothelial cells contribute to transient definitive erythroid/myeloid progenitors [28] , [29] , [30] , [31] , [32] , [33] . This haematopoietic population could also be isolated from Nkx2–5-green fluorescent protein (GFP) transgenic mouse ES cell line. As shown in Supplementary Fig. S10 , GFP + /CD41 + cells at day 4.5 and 5.5 embryoid bodies (EBs) successfully yielded erythroid, myeloid and mixed colonies, suggesting that ES-derived Nkx2–5+ cells can serve as an alternative sources for haematopoietic cells. 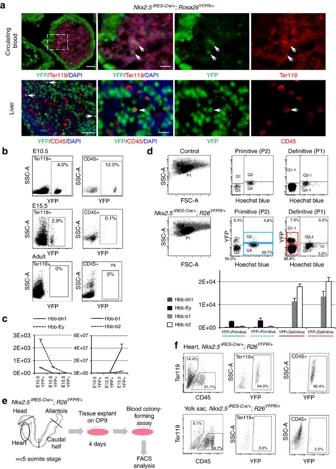Figure 4: A subset of erythroids and myeloids in the peripheral circulation arise from Nkx2–5+endocardial/endothelial cells. (a) Peripheral blood and liver inNkx2–5IRES-Cre/+; R26YFPR/+E10.5 embryo stained for YFP (green) and Ter119 (red). Double-positive cells (arrows) indicate circulating erythroids (upper panels), and CD45+cells repopulating in the liver (lower panels) are positive for YFP. Note that some endodermal cells in the liver are also labelled by YFP reporter. Scale bar, 10 μm. (b) Peripheral blood cells fromNkx2–5IRES-Cre/+; R26YFPR/+embryos at E10.5, E15.5 and adult stages were analysed for YFP, CD45 and Ter119 by FACS. Nkx2–5+cells contribute to 4.0% of Ter119+cells and 12.0% of CD45+cells at E10.5, and 2.9 and 0.1%, respectively, at E15.5. No YFP+blood cells are identified in the adult peripheral circulation. (c) Expression analyses of β-globins in Nkx2–5-derived peripheral blood at E10.5, 12.5 and 15.5 by qPCR from YFP+circulating cells ofNkx2–5IRES-Cre/+; R26YFPR/+embryos.Hbb-bh1(solid line, left) was first downregulated by E12.5 followed by downregulation ofEy(dashed line, left) by E15.5.Hbb-b1andb2were strongly upregulated by E15.5. (d) Primitive and definitive erythroids were sorted from E15.5 control andNkx2–5IRES-Cre/+; R26YFPR/+embryos based on forward and side scatters (top left panels). FACS analyses for Hoechst 33342 and YFP revealed that Nkx2–5+cells contribute to both nucleated primitive erythroids (solid blue line) and enucleated definitive erythroids (solid red line, top right panels). qPCR analysis for β-globins revealed that Nkx2–5-derived primitive and definitive erythroids dominantly express Hbb-Ey and Hbb-b1/b2, respectively (bottom panel). (e) Schematic representation of the colony-forming assay from the explant of Nkx2–5-lineage-labelled organs at pre-circulation stages. Tissues were washed in three changes of PBS and cultured on OP9 feeder for 4 days, followed by methylcellulose culture in the presence of haematopoietic growth factors. (f) FACS analysis of the colonies retrieved from Nkx2–5-lineage-labelled heart tubes and yolk sacs at pre-circulation stages. Nkx2–5-derived cells constitute 54.0% of Ter119+cells and 96.4% of CD45+cells in the colonies from the heart tubes (left), but only 3.0 and 2.2%, respectively, in those from the yolk sac (right). Figure 4: A subset of erythroids and myeloids in the peripheral circulation arise from Nkx2–5 + endocardial/endothelial cells. ( a ) Peripheral blood and liver in Nkx2 – 5 IRES-Cre/+ ; R26 YFPR/+ E10.5 embryo stained for YFP (green) and Ter119 (red). Double-positive cells (arrows) indicate circulating erythroids (upper panels), and CD45 + cells repopulating in the liver (lower panels) are positive for YFP. Note that some endodermal cells in the liver are also labelled by YFP reporter. Scale bar, 10 μm. ( b ) Peripheral blood cells from Nkx2 – 5 IRES-Cre/+ ; R26 YFPR/+ embryos at E10.5, E15.5 and adult stages were analysed for YFP, CD45 and Ter119 by FACS. Nkx2–5 + cells contribute to 4.0% of Ter119 + cells and 12.0% of CD45 + cells at E10.5, and 2.9 and 0.1%, respectively, at E15.5. No YFP + blood cells are identified in the adult peripheral circulation. ( c ) Expression analyses of β-globins in Nkx2–5-derived peripheral blood at E10.5, 12.5 and 15.5 by qPCR from YFP + circulating cells of Nkx2 – 5 IRES-Cre/+ ; R26 YFPR/+ embryos. Hbb-bh1 (solid line, left) was first downregulated by E12.5 followed by downregulation of Ey (dashed line, left) by E15.5. Hbb-b1 and b2 were strongly upregulated by E15.5. ( d ) Primitive and definitive erythroids were sorted from E15.5 control and Nkx2 – 5 IRES-Cre/+ ; R26 YFPR/+ embryos based on forward and side scatters (top left panels). FACS analyses for Hoechst 33342 and YFP revealed that Nkx2–5 + cells contribute to both nucleated primitive erythroids (solid blue line) and enucleated definitive erythroids (solid red line, top right panels). qPCR analysis for β-globins revealed that Nkx2–5-derived primitive and definitive erythroids dominantly express Hbb-Ey and Hbb-b1/b2, respectively (bottom panel). ( e ) Schematic representation of the colony-forming assay from the explant of Nkx2–5-lineage-labelled organs at pre-circulation stages. Tissues were washed in three changes of PBS and cultured on OP9 feeder for 4 days, followed by methylcellulose culture in the presence of haematopoietic growth factors. ( f ) FACS analysis of the colonies retrieved from Nkx2–5-lineage-labelled heart tubes and yolk sacs at pre-circulation stages. Nkx2–5-derived cells constitute 54.0% of Ter119 + cells and 96.4% of CD45 + cells in the colonies from the heart tubes (left), but only 3.0 and 2.2%, respectively, in those from the yolk sac (right). Full size image As Nkx2–5 lineage tracing experiments by themselves cannot distinguish Nkx2–5 + cells from endocardium or yolk sac endothelium, we examined whether Nkx2–5 + endocardial cells contribute to Ter119 + and/or CD45 + cells by pre-circulation stage explant assay using Nkx2 – 5 IRES-Cre/+ ; R26 YFPR/+ embryos ( Fig. 4e ). FACS analysis of the colonies from Nkx2 – 5 IRES-Cre/+ ; R26 YFPR/+ embryos indicates that a majority of the colonies from the heart tubes arise from Nkx2–5-positive cells. As shown in Fig. 4f , Nkx2–5-derived cells constitute 54.0% of Ter119 + cells and 96.4% of CD45 + cells in the colonies from the heart tubes, whereas only 3.0 and 2.2%, respectively, are labelled in the colonies from the yolk sac. The difference in the percentage of YFP + fractions in the heart tubes and the yolk sac further supports that the heart-derived colonies are not the result of contamination from the yolk sac during the procedure. Taken together, these data suggest that Nkx2–5 + endocardial cells give rise to transient haematopoietic progenitors for both Ter119 + erythroid and CD45 + non-erythroid cells independently from the yolk sac. Endocardial haematopoiesis is regulated by Nkx2–5 and Isl1 Specific expression of Nkx2–5 in the haemogenic endocardium leads to the question of whether or not Nkx2–5 expression is required for the haemogenic potential of the endocardium. Nkx2–5-null embryos die at around E10.5 with cardiac-looping defects, and also develop impaired angiogenesis and haematopoiesis [34] , [35] . It was previously speculated that these hemato-vascular defects are secondary to the myocardial phenotype [35] . However, the identification of Nkx2–5-positive/-derived endocardium and yolk sac endothelium raises the possibility that Nkx2–5 is directly involved in embryonic haematopoiesis. Indeed, ectopic expression of NKX2 – 5 is found in the leukaemic cells in children with T- and B-cell acute lymphoblastic leukaemia with t(5;14) translocation [36] , [37] . Given that the molecular pathways regulating oncogenesis often recapitulate aberrations of processes governing embryogenesis, these clinical observations support the idea that Nkx2–5 has a direct role during haematopoiesis. To examine the role of Nkx2–5 in endocardial haematopoiesis, we analysed Nkx2 – 5 -knockout embryos. At E9.5, Nkx2 – 5 -null hearts showed a significantly reduced number of CD41 + cells in the endocardium ( Fig. 5a , top panels). Lineage tracing of Nkx2–5-positive cells in Nkx2–5-null background ( Nkx2 – 5 Cre/Cre ; R26 YFPR/+ embryos) revealed that Nkx2–5-expressing endocardial cells were found in the endocardial layer ( Supplementary Fig. S11 ), suggesting that Nkx2–5 is required not for the migration of the haemogenic endocardial cells to the cushion but for the specification of haematopoietic progenitor cells from the endocardium. Colony-forming assays with sorted endocardial cells showed that no blood colonies are generated from Nkx2 – 5- knockout endocardium at E9.5 ( Fig. 5b , left). Furthermore, the number of Nkx2–5-derived Ter119 + cells was significantly reduced in the peripheral circulation in Nkx2–5-null background ( Nkx2 – 5 Cre/Cre ; R26 YFPR/+ embryos) at E9.5 ( Fig. 5c ). These data suggest that the expression of Nkx2–5 is required for the emergence of haematopoietic progenitors in the endocardium. 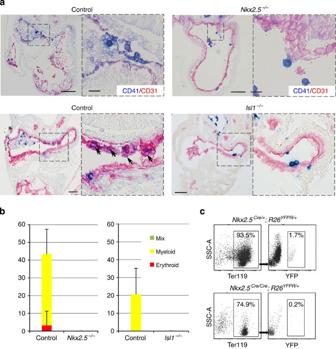Figure 5: Endocardial haematopoiesis depends on Nkx2–5 and Isl1. (a) Nkx2–5 and Isl1 mutant hearts at E9.5 stained for CD41 (blue) and CD31 (red). CD41+cells were scarce in the endocardium of Nkx2–5 or Isl1 mutant hearts. Note that Nkx2–5 mutant also develops known cardiac defects including a single ventricle with poorly developed trabeculae, open atrioventricular canal, and lack of endocardial–mesenchymal transformation in the cushion. Scale bar, 100 μm. (b) Blood colony-formation assay from FACS-purified endocardial cells. No colonies were formed from Nkx2–5-mutant endocardial cells. Data represent average of three independent experiments. Mean±s.e.m. (c) Comparison of the peripheral blood cells derived from Nkx2–5-expressing cells in Nkx2–5-null and its control backgrounds at E10.0. YFP-labelled red blood cells (Ter119+) were found less frequently (0.2%) inNkx2–5Cre/Cre; R26YFPR/+embryos compared with control littermates (1.7%), suggesting that expression of Nkx2–5 is required for the haemogenic activity of the Nkx2.5+endocardial/endothelial cellsin vivo. Figure 5: Endocardial haematopoiesis depends on Nkx2–5 and Isl1. ( a ) Nkx2–5 and Isl1 mutant hearts at E9.5 stained for CD41 (blue) and CD31 (red). CD41 + cells were scarce in the endocardium of Nkx2–5 or Isl1 mutant hearts. Note that Nkx2–5 mutant also develops known cardiac defects including a single ventricle with poorly developed trabeculae, open atrioventricular canal, and lack of endocardial–mesenchymal transformation in the cushion. Scale bar, 100 μm. ( b ) Blood colony-formation assay from FACS-purified endocardial cells. No colonies were formed from Nkx2–5-mutant endocardial cells. Data represent average of three independent experiments. Mean±s.e.m. ( c ) Comparison of the peripheral blood cells derived from Nkx2–5-expressing cells in Nkx2–5-null and its control backgrounds at E10.0. YFP-labelled red blood cells (Ter119 + ) were found less frequently (0.2%) in Nkx2 – 5 Cre/Cre ; R26 YFPR/+ embryos compared with control littermates (1.7%), suggesting that expression of Nkx2–5 is required for the haemogenic activity of the Nkx2.5 + endocardial/endothelial cells in vivo . Full size image Another key cardiac transcription factor, Isl1, is also expressed in the endocardium of outflow cushion and atria ( Supplementary Fig. S12 ) [38] , [39] . Isl1 mutants, like Nkx2 – 5 mutants, showed much less CD41 expression and no blood colony formation from the endocardium compared to control littermates at E9.5 ( Fig. 5a , bottom panels; Fig. 5b , right). These data suggest that Isl1 is also required for the emergence of CD41 + cells in the endocardium. In conclusion, we have demonstrated that Nkx2–5-positive subset of the endocardium and yolk sac endothelium gives rise to progenitors for transient definitive haematopoiesis that contribute to circulating erythroid/myeloid cells until late gestational stages via an Nkx2–5- and Isl1-dependent mechanism. Given that the endocardial cells may be heterogeneous in their origins [40] , [41] , [42] , [43] , an intriguing possibility is that the haemogenic endocardial cells are derived from multipotent Flk1/Isl1/Nkx2–5-positive cardiovascular progenitors [12] through endocardial intermediates. Indeed, haemogenic endocardial cells express all these markers ( Fig. 3 ; Supplementary Fig. S12 ) [38] , [39] , and early cardiac progenitors express multiple haematopoietic transcription factors [12] , [13] . Alternative possibility is that yolk sac-derived Runx1 + precursors contribute to haemogenic endocardial cells as in the dorsal aorta [44] . The identification of haemogenic endocardial cells in this study potentially adds a haematopoietic component into the cardiovascular lineage tree and places Nkx2–5 at the centre of diverse cardio-vasculo-haematopoietic lineages. Finally, it leads to a better understanding of the origins and roles of transient definitive haematopoiesis during embryogenesis and leukemogenesis. Mouse models Genetically modified Nkx2–5-null, Nkx2–5-IRES-Cre, Nkx2–5-Cre, NCX1-null, Isl1-null, Runx1-rd and Runx1-lz mouse lines are described previously [22] , [25] , [45] , [46] , [47] , [48] , [49] . Animals were maintained in accordance with the guidelines of the UCLA Animal Research Committee. Preparation of frozen tissue sections Mouse embryos were isolated in cold PBS and fixed in 4% paraformaldehyde for 2–3 h, followed by equilibration in 30% sucrose in PBS solution overnight. The tissues were placed in 1:1 30% sucrose/OCT (Tissue-Tek, Electron Microscopy Sciences) solution for 1–2 h, in 100% OCT compound for 1 h at 4 °C, and embedded in 100% OCT compound, carefully oriented in Cryomolds (Ted Pella). The blocks were immediately frozen on dry ice with isopropanol and stored at −80 °C. The sections were cut 7–10 μm with a Leica CM3050 S cryostat. The following primary antibodies were used: rat CD41 (1:50, BD PharMingen), Phospho-Histone 3 (1:200, Millipore), Ter119 (1:50 eBioscience) and PECAM-1/CD31 (1:200, BD PharMingen) were used on fixed frozen sections. Tyramide amplification (Invitrogen) was applied to CD41 and Ter119 stainings. The following secondary antibodies were used: biotinylated IgG antibodies (Vector Laboratories) for colorimetric staining and Alexa Fluor 488 (green), Alexa Fluor 594 (red)-conjugated secondary antibodies specific to the appropriate species were used (1:500; Invitrogen) for fluorescent staining. Sections were mounted with antifade mounting medium with DAPI (Invitrogen), and analysed by using AxioImager D1 (Carl Zeiss Microimaging Inc.). Electron microscopic analysis Tissues were fixed in 1% glutaraldehyde, 4% paraformaldehyde in PBS and washed. After post-fixation in 1% OsO4 in PB for 1 h, the tissues were dehydrated in a graded series of ethanol, treated with propylene oxide and embedded in Eponate 12 (Ted Pella). Approximately 60–70-nm-thick sections were cut on a Reichert–Jung Ultracut E ultramicrotome and picked up on formvar-coated copper grids. The sections were stained with uranyl acetate and Reynolds lead citrate, and examined on a JEOL 100CX electron microscope at 80 kV. Flow cytometry for sorting cells of mouse embryonic tissues We harvested tissues from mouse embryos of several developmental stages (E9.5–10.5). Isolated tissues were washed three times and incubated at 37 °C in a dissociation enzyme solution with occasinal pipetting to a single-cell suspension. The enzyme solution contained 1% Penicillin/Streptomycin (Invitrogen, 15140-122), 10% fetal bovine serum (Hyclone), collagenase 2 mg ml −1 (Worthington, CLS-2), dispase 0.25 mg ml −1 (Gibco, 17105-041), DNAase I (Invitrogen) in PBS. The cells were analysed and sorted by a BD FACSAria with the following rat anti-monoclonal antibodies: CD41-PE-Cy7 (eBioscience), CD45APC (BD Pharmingen), Ter119 (eBioscience), ckit-APC-Cy7 (Biolegend), CD31-PE (BD Pharmingen). 7-AAD (7-amino-actinomycinD, BD Biosciences) staining was used to exclude non-viable cells. Haematopoietic colony-forming assays Sorted cells, as described above, were cultured on OP9 stromal cells for 4 days in 48-well plates in 500 μl of α-MEM (Gibco/Invitrogen) containing 20% fetal bovine serum (Hyclone), 1% penicillin/streptomycin and supplemented with stem cell factor (SCF, 50 ng ml −1 ), interleukin-3 (IL-3, 5 ng ml −1 ), IL-6 (5 ng ml −1 ), thrombopoietin (5 ng ml −1 ) and Flt-3 ligand (Flt-3L, 10 ng ml −1 ). The cells were then dissociated mechanically from stroma by transfer pipette and filtered to remove the stromal cells (celltreck). The filtered cells were transferred into 1.5 ml methylcellulose with SCF, IL-6, IL-3 and EPO (MethoCult 3434, Stem Cell Technologies) supplemented with thrombopoietin (5 ng ml −1 ) to determine multilineage potential. Colonies were scored 7–10 days later. Embryonic stem cell culture Nkx2–5-EmGFP ES cell line [50] was maintained on irradiated feeder. After the differential plating of feeder for 45 min on gelatin-coated dish, 100 non-adherent cells were collected in 10 μl of IMDM-based hanging drop containing 15% FBS, MTG, hTransferrin, ascorbic acid (25 μg ml −1 ), hBMP (45 ng ml −1 ), mSCF (50 ng ml −1 ) and mVEGF (10 ng ml −1 ). EBs in hanging drops were plated on day 2 on ultra low attachment plate, and cultured in the same media until the FACS sorting. Organ explant culture Fetal organs were dissected out, washed three times and mechanically dissociated to small pieces. They were cocultured on mouse OP9 stromal cells in the same media used for the haematopoietic colony-forming assay. After 4 days of culture, they were transferred into methylcellulose in the same way as described in the haematopoietic colony-forming assay method. Gene expression analysis by microarray RNeasy Micro Kit (Qiagen) was used to isolate total RNA from sorted cells from biological replicates of each cell population. RNA amplified by Nugen kit was hybridized on Affymetrix MOE 430 2.0 mouse gene expression microarrays. We used the R package Limma [51] provided through the open source project Bioconductor (version 2.7) [52] for assessing differential expression. To obtain a final list of differentially expressed genes, thresholds for selecting significant genes were set at a relative fold difference >2-fold and P -value <0.01 on the list of probe sets reported by Limma . To calculate absolute mRNA expression levels, we used the RMA (Robust Multiarray Averaging [53] ) method provided through R library Affy to obtain background adjusted, quantile normalized and probe level data summarized values for all probe sets. For genes with multiple probe sets, in order to avoid overcounting, we chose the probe set with the lowest P -value. Official gene symbols for probe sets were obtained using the Bioconductor annotation database mouse4302.db. Differentially up- and downregulated gene sets were uploaded into the online DAVID interface to identify statistically significantly over-represented gene ontology biological process categories. We used the MAS5.0 algorithm [54] through the Affy for calculating phorbol myristate acetate detection calls for each array sample. The algorithm employs a signed rank test to consider the significance of the difference between the PM (Perfect Match) and MM (MisMatch) values for each probeset and returns a detection P -value that is used to flag a transcript as ‘Present’, ‘Marginal’ or ‘Absent’ (P/M/A). Gene expression analysis by quantitative reverse-transcriptase PCR RNA was extracted from the sorted cells using with RNeasy Micro Kit (Qiagen). RNA was reverse-transcribed into complementary DNA using the iScript cDNA synthesis kit (BioRad). Quantitative reverse-transcriptase PCR was performed using Lightcycler 480 SYBR Green I (Roche Applied Science). Forward and reverse primer sequences are as follows: Hbb-bh1 ; 5′-aggcagctatcacaagcatctg-3′, 5′-aacttgtcaaagaatctctgagtccat-3′ Hbb-Ey ; 5′-caagctacatgtggatcctgagaa-3′, 5′-tgccgaagtgactagccaaa-3′ Hbb-b1 ; 5′-cgtttgcttctgattctgttg-3′, 5′-ctagatgcccaaaggtcttc-3′ Hbb-b2 ; 5′-aaaggtgaaccccgatgaag-3′, 5′-tgtgcatagacaatagcaga-3′ Gapdh ; 5′-gaagggcatcttgggctacac-3′, 5′-gcagcgaactttattgatggtatt-3′ Accession Codes: All original microarray data have been deposited in NCBI’s Gene Expression Omnibus under accession number GSE40260 . How to cite this article: Nakano, H. et al . Haemogenic endocardium contributes to transient definitive haematopoiesis. Nat. Commun. 4:1564 doi: 10.1038/ncomms2569 (2013).